Hopping transport and the Hall effect near the insulator–metal transition in electrochemically gated poly(3-hexylthiophene) transistors Despite 35 years of investigation, much remains to be understood regarding charge transport in semiconducting polymers, including the ultimate limits on their conductivity. Recently developed ion gel gating techniques provide a unique opportunity to study such issues at very high charge carrier density. Here we have probed the benchmark polymer semiconductor poly(3-hexylthiophene) at electrochemically induced three-dimensional hole densities approaching 10 21 cm −3 (up to 0.2 holes per monomer). Analysis of the hopping conduction reveals a remarkable phenomenon where wavefunction delocalization and Coulomb gap collapse are disrupted by doping-induced disorder, suppressing the insulator–metal transition, even at these extreme charge densities. Nevertheless, at the highest dopings, we observe, for the first time in a polymer transistor, a clear Hall effect with the expected field, temperature and gate voltage dependencies. The data indicate that at such mobilities (~0.8 cm 2 V −1 s −1 ), despite the extensive disorder, these polymers lie close to a regime of truly diffusive band-like transport. Despite a 35-year effort, semiconducting polymers continue to provide serious challenges to our understanding of charge transport in solids [1] , [2] , [3] , [4] . Elusive issues include the non-trivial influence of the multiple sources of disorder (for example, semi-crystallinity, paracrystallinity and nanoscale inhomogeneity [1] , [2] , [3] , [4] , [5] , [6] , [7] ), the elucidation of the important hopping mechanisms [1] , [2] , [3] , [4] , [7] , [8] , [9] , [10] , the effects of charge carrier–lattice interactions [3] , [4] and the identification of the ultimate limits on conductivity and mobility [1] , [2] , [3] , [4] , [5] , [6] , [11] . The latter is particularly important as, in addition to being of considerable fundamental interest the upper limits on conductivity and mobility also limit device performance (for example, transistor output current and operating frequency). In this context it is important to note that in the vast majority of cases these semiconducting polymers populate the insulating side of the Mott–Anderson insulator–metal transition, where transport occurs by thermally assisted hopping between localized electronic states (for example, refs 1 , 2 , 3 , 4 and 7 , 8 , 9 ). In fact, it is only in a limited number of cases (for example, free-standing thick films of semiconducting polymers such as polyaniline (for example, refs 11 and 12 ) or polypyrrole (for example, ref. 13 )) that chemical doping can delocalize carrier wavefunctions to the point of inducing an insulator–metal transition to a state with finite conductivity as T →0, or even entering the weakly localized regime beyond it [12] , [13] . It is currently unclear whether a metallic state is possible only in certain semiconducting polymers, or whether efficacy of chemical doping, or minimization of disorder, limit delocalization of the charge carriers. In addition, and in contrast to lower disorder organic conductors such as small molecule systems, the anticipated crossover from non-adiabatic hopping to diffusive band transport with increasing carrier density has not yet been observed in semiconducting polymers. It has been argued that such a crossover is expected when the mobility reaches a quasi-universal value of ~1 cm 2 V −1 s −1 ( [4] ). In one of the most important recent advances in organic electronics, this value has now been surpassed in electrostatically gated surface layers of single-crystal small molecule semiconductors such as rubrene (for example, refs 14 and 15 ). Electrostatic gating in the field-effect transistor geometry is ideal for such studies, as it enables wide-range tuning of the carrier density in a single sample [16] . A clear crossover to band transport has indeed been detected in such devices, via observation of a phonon-limited temperature dependence of the mobility, a robust Hall effect, and equivalence of the Hall mobility and the mobility extracted from gate voltage-dependent measurements [14] , [15] . Semiconducting polymers, perhaps unsurprisingly given their lower crystallinity, low bandwidth and greater disorder, lag somewhat behind. Although the mobilities of benchmark semiconducting polymers such as poly(3-hexylthiophene; P3HT) are now at, or are approaching, the 1 cm 2 V −1 s −1 threshold in thin film transistors [17] , [18] , no phonon-limited mobility has been observed and no Hall effect has been reported. In this work we exploit the recent developments with ionic liquid/gel gating techniques in thin film transistors to study electrochemically doped P3HT at three-dimensional (3D) hole densities up to 10 21 cm −3 , that is, 0.2 holes per monomer. An insulator–metal transition does not take place even at these extreme densities, an effect that can be traced back via detailed analysis of the variable-range hopping (VRH) conduction to doping-induced disorder, preventing carrier wavefunction delocalization and Coulomb gap collapse. The results thus point to a serious potential limitation of electrochemical doping in such systems. Nevertheless, at the highest dopings and temperatures, we observe for the first time in a semiconducting polymer thin film transistor, a robust Hall signal with expected field, temperature and gate voltage dependencies. The data suggest that at these mobilities (~0.8 cm 2 V −1 s −1 ), despite the extensive disorder, such solution-processed films lie close to a regime of truly diffusive band-like transport. Electrochemical thin film transistors A schematic of the device studied (see Methods section for synthesis details) is shown in Fig. 1a . An optical micrograph and further characterization details are provided in Supplementary Fig. S1 . In essence, the device is a four-terminal bottom-contacted van der Pauw geometry P3HT thin film transistor, gated electrochemically using an ion gel based on an ionic liquid (1-ethyl-3-methylimidazolium bis(trifluoro-methylsulfonyl) imide ((EMIM)(TFSI))) and a triblock copolymer (poly(styrene- b -methylmethacrylate- b -styrene; PS-PMMA-PS)) [19] , [20] , [21] . Such ionic liquids and gels have been used recently to electrostatically induce two-dimensional charge densities ~10 14 cm −2 in a variety of materials (for example, refs 22 , 23 , 24 , 25 ). In the case of semi-crystalline semiconducting polymers such as P3HT, the open structure results in deep penetration of the dopant ions, providing uniform 3D electrochemical doping ( Fig. 1b ) [21] , [26] . That the P3HT thickness employed here (60 nm) can be safely assumed to be in the 3D doping limit is well established [21] , [26] . Although quantification of P3HT crystallinity remains a challenge, it is generally regarded to be quite low [6] , and heavy electrochemical doping is expected to further reduce it. We thus view the system as predominantly amorphous. However, the P3HT used here is of a high-enough molecular weight ( M n =23 kDa, see Methods) to lie on the saturation region of the mobility versus the M n curve [27] , approaching 1 cm 2 V −1 s −1 in annealed devices. 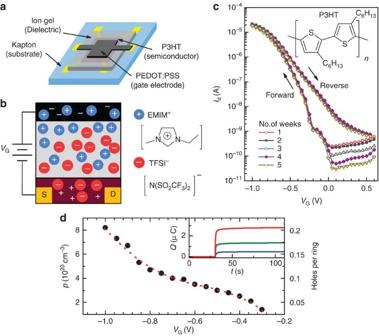Figure 1: Schematics andI–Vcharacteristics of electrochemically gated P3HT transistors. (a) Schematic of the van der Pauw geometry device structure (channel size is 500 μm × 500 μm). An optical image of an actual device is shown inSupplementary Fig. S1. (b) Schematic of charge injection into the polymer semiconductor. The top layer (black) is the gate electrode, the middle layer (grey) is the ion gel and the bottom layer (maroon) is the polymer semiconductor. Simple ‘+’ and ‘−’ symbols are used for electronic charge carriers, and blue and red symbols are used for ions. The chemical structures of EMIM+and TFSI−are shown on the right. (c) Drain current (Id) versus gate voltage (VG) at 280 K measured 1 week apart for 5 consecutive weeks.VGwas swept at 50 mV s−1. The inset shows the chemical structure of P3HT. (d) Gate voltage (VG) dependence of the hole density (p). The right axis shows the conversion to holes per thiophene ring. The inset shows accumulated charge (Q, integrated from the gate current) versus time. The top (red), middle (green) and bottom (blue) curves are for −1.00, −0.65 and −0.30 V, respectively. Figure 1: Schematics and I–V characteristics of electrochemically gated P3HT transistors. ( a ) Schematic of the van der Pauw geometry device structure (channel size is 500 μm × 500 μm). An optical image of an actual device is shown in Supplementary Fig. S1 . ( b ) Schematic of charge injection into the polymer semiconductor. The top layer (black) is the gate electrode, the middle layer (grey) is the ion gel and the bottom layer (maroon) is the polymer semiconductor. Simple ‘+’ and ‘−’ symbols are used for electronic charge carriers, and blue and red symbols are used for ions. The chemical structures of EMIM + and TFSI − are shown on the right. ( c ) Drain current ( I d ) versus gate voltage ( V G ) at 280 K measured 1 week apart for 5 consecutive weeks. V G was swept at 50 mV s −1 . The inset shows the chemical structure of P3HT. ( d ) Gate voltage ( V G ) dependence of the hole density ( p ). The right axis shows the conversion to holes per thiophene ring. The inset shows accumulated charge ( Q , integrated from the gate current) versus time. The top (red), middle (green) and bottom (blue) curves are for −1.00, −0.65 and −0.30 V, respectively. Full size image Critical to the success of this study, which involves cryogenic transport measurements over a wide carrier density range on a single device, was the development of device designs and fabrication methods, resulting in robust, repeatable transport properties over long time periods and multiple thermal cycles. This is illustrated in Fig. 1c , which shows 280 K transfer curves (that is, source-drain current ( I d ) versus gate voltage ( V G ) plots) for a single device over a 5-week period and >30 thermal cycles. The device has on/off ratios approaching 10 6 , threshold voltages around −0.5 V and modest V G hysteresis. Bias-stress effects are negligible, enabling drift-free isothermal magnetic field sweeps for facile measurement of magnetoresistance and the Hall effect. Aside from the decrease in off current, which we ascribe to a gradual decrease in oxygen content, no significant change in performance with time is observed. As a simple measure of the total injected charge density, Q , the gate current during charging was integrated over long times (for example, see inset in Fig. 1d at V G =−0.30, −0.65 and −1.00 V). The main panel of Fig. 1d shows the result of repeating this procedure from −0.3 to −1.0 V at 280 K, the −1.0 V upper limit being set by the irreversible decrease in conductivity that occurs beyond this voltage with this particular ionic liquid. Note that this irreversible conductivity decrease at high | V G | is not universal. In transistors based on some organic conductor/ionic liquid (or gel) combinations, reversible conductivity decreases are observed at high | V G | (for example, ref. 26 ). The highest hole densities ( p ) estimated are around 8 × 10 20 cm −3 , corresponding (right axis) to 0.2 holes per thiophene ring. In the main set of experiments presented here, the devices are first electrochemically gated to the desired V G , the gate current integrated and then cooled below the freezing temperature of the ion gel (~220 K) to fix p . All subsequent measurements are made in the Ohmic response regime as shown in Supplementary Fig. S2 and discussed in the Methods section. Hopping transport By varying V G from −0.3 to −1.0 V in 0.05 V increments, we measured the temperature dependence of the resistivity, ρ , at 15 distinct p values between ~10 20 and 10 21 cm −3 in a single electrochemical device. The data are plotted as ρ (log scale) versus T in Supplementary Fig. S2(c) , and as ρ (log scale) versus T − 1/2 and T − 1/4 in Fig. 2a , down to 1.5 K. Although the 250 K resistivity can be decreased by well over three orders of magnitude to values as low as 12 mΩ cm (a conductivity of 83 scm −1 ), d ρ /d T remains negative even at p =8 × 10 21 cm −3 . Indeed, the conductivity does not extrapolate to finite values as T →0, indicating that an insulator–metal transition is absent. Rather, we shall show that Fig. 2a–c demonstrate conclusively that the mechanism of conduction is actually VRH. As shown in Fig. 2a , log( ρ ) is linear in T −1/2 over the whole accessible T range for p <6 × 10 20 cm −3 . For p >6 × 10 20 cm −3 , log( ρ ) is linear in T −1/2 only at low T ( Fig. 2a ), being instead linear in T −1/4 at high T ( Fig. 2b ). Verification of these deduced T exponents, via an unbiased quantitative analysis, was achieved via the logarithmic derivative method, where w =–d(ln ρ )/d(ln T ) is plotted as a function of ln T to linearize ρ = ρ 0 exp ( T 0 / T ) x , yielding − x directly from the slope. As can be seen from Fig. 2c , this process confirms x ~0.5 over the whole T range for low p (<6 × 10 20 cm −3 ), and a T -dependent crossover from x ~0.5 to x ~0.25 at high p (>6 × 10 20 cm −3 ). Critically, and as returned to below, at the highest p values only, the data of Fig. 2c also suggest the existence of a crossover to a third regime (arrow in Fig. 2c ) at high T . 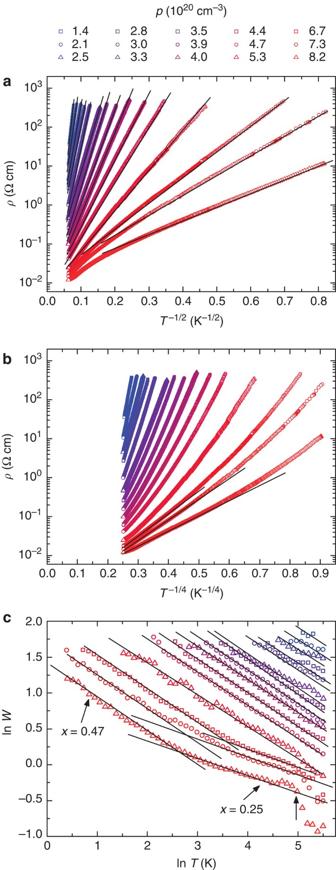Figure 2: Temperature dependence of the zero magnetic field resistivity (ρ). (a) lnρversusT−1/2for 15 distinct gate-induced carrier densities (in units of 1020cm−3), in a single device. The solid lines are straight line guides to the eye. (b) lnρversusT−1/4for the same 15 carrier densities. The solid lines are straight line guides to the eye. (c) lnWversus lnTplot for the same 15 carrier densities, whereW, the logarithmic derivative, is defined as –d(lnρ)/d(lnT). The solid lines correspond tox~−0.5 andx=−0.25. The vertical arrow indicates the departure from hopping behaviour. The symbol key shown at the top of panelaapplies to panelsa–c. Figure 2: Temperature dependence of the zero magnetic field resistivity ( ρ ). ( a ) ln ρ versus T −1/2 for 15 distinct gate-induced carrier densities (in units of 10 20 cm −3 ), in a single device. The solid lines are straight line guides to the eye. ( b ) ln ρ versus T −1/4 for the same 15 carrier densities. The solid lines are straight line guides to the eye. ( c ) ln W versus ln T plot for the same 15 carrier densities, where W , the logarithmic derivative, is defined as – d (ln ρ )/ d (ln T ). The solid lines correspond to x ~−0.5 and x =−0.25. The vertical arrow indicates the departure from hopping behaviour. The symbol key shown at the top of panel a applies to panels a – c . Full size image Given the 3D nature of this system, the T − 1/4 behaviour at relatively high T can be readily identified as Mott VRH, where ρ = ρ Mott exp ( T Mott / T ) 1/4 , with ρ Mott being the T →∞ value of ρ ( T ) and T Mott being a characteristic temperature [28] . In general, T Mott =18/ k B L C 3 N ( E F ), where L C is the localization length (that is, the decay length of the exponentially localized wavefunctions) and N ( E F ) is the density of states at the Fermi level, E F (ref. 28 ). The T −1/2 behaviour, however, could be interpreted in a number of ways, particularly conventional Efros–Shklovskii (ES) VRH [29] or inter-cluster hopping [30] . In conventional ES VRH, Coulomb interaction effects lead to a soft-gapped density of states around E F giving ρ = ρ ES exp ( T ES / T ) 1/2 , where T ES =2.8 e 2 / κk B L C , and κ is the dielectric constant [29] . A similar T dependence can, however, also be obtained from thermally assisted tunnelling between nanoscopic conductive regions in a more insulating matrix, due to the Coulomb penalty associated with single carrier charging [30] . Such models have been adapted to semiconducting polymers [8] and claims of observation of this mechanism have been made [9] . We thus performed additional analyses and measurements to clarify the origin of the T −1/2 behaviour. The first of these analyses is displayed in the inset to Fig. 3a , which compares the observed temperature of crossover between T −1/2 and T −1/4 regimes, and the predicted crossover temperature, assuming ES VRH. The latter occurs at 16 T ES 2 / T Mott (refs 9 , 31 ) and, as demonstrated by the straight line fit with slope 1, the agreement with the experiment is very good, strongly supporting interpretation as conventional ES VRH. Further evidence is provided by magnetoresistance measurements with magnetic field ( H ) perpendicular to the device plane, where large positive magnetoresistance is expected due to field-induced suppression of wavefunction overlap. In the weak field limit, ES VRH is expected to result in ln( ρ ( H )/ ρ (0))= t ( e / ch ) 2 H 2 L C 4 ( T / T 0 ) −1.5 , with t =0.0015 ( [29] ). Representative data at p =8.2 × 10 21 cm −3 are presented as a function of T and H in Fig. 3a , respectively. 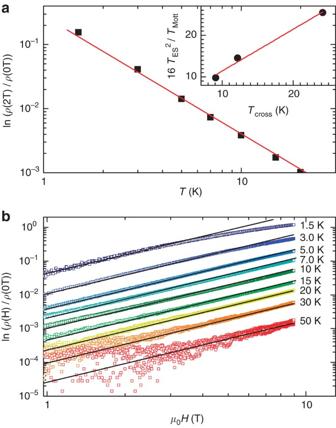Figure 3: Magnetoresistance. (a) Log–log plot of ln(ρ(μ0H=2T)/ρ(0)) versusTatp=8.2 × 1021cm−3.His the applied magnetic field. The solid line has a slope of −1.8. The inset shows the predicted crossover temperature from ES to Mott VRH (that is, 16TES2/TMott) versus the observed crossover temperature,Tcross. The solid line is a linear fit with a slope of 1.0. (b) Log–log plot of ln(ρ(H)/ρ(0)) versusμ0Hfor temperatures from 1.5 to 50 K atp=8.2 × 1021cm−3. The solid lines have slopes of 1.9. Figure 3b confirms the existence of large positive magnetoresistance increasing rapidly with decreasing T , with a ln( ρ ( H )/ ρ (0)) ∝ H 1.9 dependence, in good agreement with theory. Figure 3a reveals ln( ρ (2 T)/ ρ (0)) ∝ T − 1.8 , again in reasonable agreement with theory for ES VRH. Indeed, with the exception of the small negative deviations from the predicted H dependence at the lowest T (which are quite common but do not correspond to simple estimates for the crossover from the weak- to high-field limits), we conclude that the ES VRH accounts quantitatively for all aspects of our low T data. We interpret the apparent adherence to conventional models of VRH, with no modifications for charge carrier–lattice or polaronic effects, as evidence that in the majority of the parameter space studied here we are in a regime of strongly non-adiabatic transport with hopping energies significantly smaller than polaron transport or formation energies. As discussed in more detail below, we believe that the deviations from hopping behaviour at high T and p in Fig. 2c signal a crossover to a more adiabatic regime where polaronic effects may be more important. Figure 3: Magnetoresistance. ( a ) Log–log plot of ln( ρ ( μ 0 H =2T)/ ρ (0)) versus T at p =8.2 × 10 21 cm −3 . H is the applied magnetic field. The solid line has a slope of −1.8. The inset shows the predicted crossover temperature from ES to Mott VRH (that is, 16 T ES 2 /T Mott ) versus the observed crossover temperature, T cross . The solid line is a linear fit with a slope of 1.0. ( b ) Log–log plot of ln( ρ ( H )/ ρ (0)) versus μ 0 H for temperatures from 1.5 to 50 K at p =8.2 × 10 21 cm −3 . The solid lines have slopes of 1.9. Full size image It is natural to question why the crossover from Mott to ES VRH occurs at such high T . In inorganic semiconductors, for instance, this crossover is observed below 1 K (for example, ref. 32 ), when thermal fluctuations are lowered to the point that the Coulomb gap is no longer smeared. Insight into this is provided by Fig. 4a , which plots T ES ( p ), the right axis showing the conversion (see Supplementary Methods ) to Δ C , the Coulomb gap width. The values (up to 100 meV at the lowest p ) are large cf. conventional inorganic semiconductors, an observation that was previously used to argue for some form of inter-cluster hopping over ES VRH [9] . As discussed above, we believe the evidence for ES VRH is overwhelming here; we rather interpret the high T ES and Δ C in terms of the low κ values in semiconducting polymers via Δ C = e 3 N ( E F ) 1/2 / κ 3/2 . There are, in fact, obvious parallels with the relative importance of excitonic effects in organic and inorganic semiconductors. 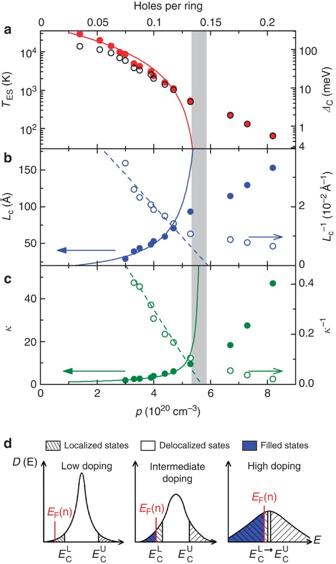Figure 4: The approach to the insulator–metal transition. Panelsa–cshow the doping dependence of the characteristic temperature of the ES hopping (TES), the localization length (LC) and the dielectric constant (ε). These quantities are plotted as solid symbols, corresponding to the left axes. The open symbols (corresponding to the right axes) show, respectively, the conversion to the Coulomb gap (ΔC) (a), and the inverse localization length (b) and dielectric constant (c). The top axis shows the conversion to holes per thiophene ring. The solid (dashed) lines ina–care fits toTES,LC(LC−1) andε(ε−1) forp<5 × 1020cm−3. The fitting equations (parameters) areTES=T0(1−p/pc)2(T0=47,000 K andpc=5.5 × 1020cm−3),LC=LC0(1−p/pc)−1(LCO=16 Å andpc=5.9 × 1020cm−3) andε=ε0(1−p/pc)−1(ε0=1.3 andpc=5.7 × 1020cm−3). The grey shaded region represents the vicinity of the hypothetical insulator–metal transition in the absence of doping-induced disorder. (d) Schematic of the evolution of the HOMO (highest occupied molecular orbital) density of states with electrochemical doping.EF(p) is the doping-dependent Fermi level, andECL,Uare the mobility edges in the upper and lower region of the HOMO. Figure 4: The approach to the insulator–metal transition. Panels a – c show the doping dependence of the characteristic temperature of the ES hopping ( T ES ), the localization length ( L C ) and the dielectric constant ( ε ). These quantities are plotted as solid symbols, corresponding to the left axes. The open symbols (corresponding to the right axes) show, respectively, the conversion to the Coulomb gap ( Δ C ) ( a ), and the inverse localization length ( b ) and dielectric constant ( c ). The top axis shows the conversion to holes per thiophene ring. The solid (dashed) lines in a – c are fits to T ES , L C ( L C −1 ) and ε ( ε −1 ) for p <5 × 10 20 cm −3 . The fitting equations (parameters) are T ES = T 0 (1− p / p c ) 2 ( T 0 =47,000 K and p c =5.5 × 10 20 cm −3 ), L C = L C0 (1− p / p c ) −1 ( L CO =16 Å and p c =5.9 × 10 20 cm −3 ) and ε = ε 0 (1− p / p c ) −1 ( ε 0 =1.3 and p c =5.7 × 10 20 cm −3 ). The grey shaded region represents the vicinity of the hypothetical insulator–metal transition in the absence of doping-induced disorder. ( d ) Schematic of the evolution of the HOMO (highest occupied molecular orbital) density of states with electrochemical doping. E F ( p ) is the doping-dependent Fermi level, and E C L,U are the mobility edges in the upper and lower region of the HOMO. Full size image Approach to the insulator–metal transition In Fig. 4a–c , we plot the p dependence of the other parameters extracted from the VRH analysis of ρ ( T , H ). Figure 4b shows L C ( p ) extracted from magnetoresistance data, using the formula provided above. Note that very similar L C values are obtained regardless of whether we fit the T dependence at fixed H ( Fig. 3a ), or the H dependence at fixed T ( Fig. 3b ). Figure 4c then plots κ ( p ) deduced from T ES ( p ) and L C ( p ) via T ES =2.8 e 2 / κk B L C . Although the qualitative behaviour is as expected ( T ES drops with p due to increases in L C and κ ), quantitatively these results lie far from simple expectations. Specifically, the expected divergences in L C and κ with increasing p as the insulator–metal transition is approached, should follow the scaling theory of electron localization, that is, L C = L C0 (1− p / p c ) −ν and κ = κ 0 (1− p / p c ) −α , where p c is the critical carrier density for the insulator–metal transition, and L C0 and κ 0 are the undoped values of L C and κ [28] . This leads to the collapse of the Coulomb gap according to T ES = T ES0 (1− p / p c ) ν+α . Although controversy remains over the precise values of the exponents, ν is often found to be unity, whereas α is often 1 or 2 (refs 28 and 29 ). It is abundantly clear from Fig. 4a–c that these scaling forms are violated in our case. L C and κ are anomalously weakly p -dependent, no divergence taking place, no collapse in Δ C occurring and, thus, no insulator–metal transition being induced. As shown in Supplementary Fig. S3 , these V G dependencies of T ES and L C , and indeed all other transport parameters, are robust, being observed in multiple devices. Further insight is obtained by fitting only the low p region ( p <5 × 10 20 cm −3 ) of T ES ( p ), L C ( p ) and κ ( p ) to the expected scaling forms. Purely for the purpose of demonstration, we fix ν and α at 1, at which point we find that reasonable fits to all three quantities can be obtained with a single p c value around 5.7 × 10 20 cm −3 . This is illustrated by the right axes of Fig. 4b , which plot L C −1 ( p ) and κ −1 ( p ), yielding reasonable linear fits for p <5 × 10 20 cm −3 . In essence, at low doping L C and κ increase in a manner consistent with the scaling theory, and a hypothetical p c ~5.7 × 10 20 cm −3 (0.14 dopant ions per monomer). Before this doping value is reached, however, adherence to scaling is lost, L C and κ become weakly p -dependent, no divergences occur and, thus, the insulator–metal transition does not take place. Note that the low p fits also yield perfectly reasonable values for L C0 and κ 0 ; we find L C0 ~15 Å, corresponding to ~3 thiophene rings, and κ 0 ~1.5, reasonably close to the accepted value [33] . We propose that the key concept to understand the anomalous doping dependence of the parameters shown in Fig. 4a–c is electrochemical doping-induced disorder. The p value at which adherence to the expected scaling forms is lost corresponds to >0.1 dopant ions per monomer. We hypothesize that at these extreme electrochemical doping levels, the forced insertion of dopant ions into the P3HT leads to substantial increases in disorder, likely to the point of additional loss in crystallinity. This competes with the increase in hole density, preventing divergence of L C and κ , and thus collapse of Δ C . In essence, p c becomes doping-dependent. To further illustrate this concept, Fig. 4d provides sketches of the available density of states, D ( E ), in the narrow valence band of P3HT at low (<5 × 10 20 cm −3 ), intermediate (~5 × 10 20 cm −3 ) and high p (>5 × 10 20 cm −3 ). We consider the situation where at low p some delocalized states exist near the middle of the band, separated from the exponentially localized ones in the band tails by the lower and upper mobility edges, E C L and E C U . As p is increased, E F ( p ) rises, L C and κ begin to diverge in accordance with the scaling theory, Δ C falls and an insulator–metal transition is anticipated as E F ( p )→ E C L . However, the increasing disorder associated with the high levels of electrochemical doping required to reach this point leads to additional Anderson localization and an increase in E C L with p , thus suppressing the insulator–metal transition. As is hopefully clear from the illustration of the high p regime in Fig. 4d , it is thus unclear whether an insulator–metal transition is possible with this type of doping, that is, whether E F can be increased sufficiently before the region of delocalized states between E C L and E C U vanishes. This may in fact be directly relevant to the puzzling recent observations of reversible decreases in conductance at high | V G | in similar devices [26] . Hall effect Although the insulator–metal transition is not reached in our devices, the distinct departure from hopping behaviour in ρ ( T ) above ~150 K at the highest p values ( Fig. 2c ) raises the possibility of a departure from the non-adiabatic hopping regime, potentially to a regime of diffusive transport. We thus searched for a Hall effect in the high p , high T region. Although the Hall effect has been reported sporadically in bulk semiconducting polymer samples on the metallic side of the insulator–metal transition [11] , [34] , its detection in thin film transistors and on the insulating side of the transition has traditionally been thwarted by low mobilities and high contact resistances. In our case, the mobility values are comparable to the best reported in P3HT thin film transistors (approaching 1 cm 2 V −1 s −1 ), and contact resistances are minimized by electrochemical doping [35] . As demonstrated by the representative 190 K data shown in the inset to Fig. 5 (more data are provided in Supplementary Figs S4 and S5 ), a robust Hall effect is indeed observed at the three highest | V G | values. The Hall resistivity ( ρ Hall ) has the expected response to sign reversal of the current and magnetic field, is linear in H , and yields a positive Hall coefficient ( R H ), consistent with hole transport (see Supplementary Fig. S5 ). It must be emphasized that R H increases with increasing | V G |. We believe this signals the emergence from the hopping regime (where the Hall effect is unmeasurably small) and the onset of a crossover towards diffusive transport. The extent to which this crossover is complete is clarified by the data in the main panel of Fig. 5 , where the p dependence of the mobility, μ ( p )=1/ peρ ( p ), is plotted using p values extracted both from our standard integration of the gate current ( μ Gate ) and from the Hall effect ( μ Hall ). For this purpose, the Hall effect is assumed to be dominated by a single carrier type; the observed linearity with magnetic field is important in this regard. A rapid, three order of magnitude increase in μ Gate is observed on increasing p from 1 to 5 × 10 20 cm −3 , followed by a much slower increase at the highest p . The μ Hall on the other hand is first detected around 6.5 × 10 20 cm −3 (0.05 cm 2 V −1 s −1 ), increasing relatively quickly at higher p . We find μ Hall ( p )< μ Gate ( p ) at all p , although the two values converge asymptotically in the high p limit. This again reflects the emergence from the non-adiabatic hopping regime (where R H is very small) and the crossover towards diffusive transport where μ Hall ( p )~ μ Gate ( p ) is expected. That this crossover is not complete is further clarified by μ Hall ( T ) (see Supplementary Fig. S4 , at V G =−1 V), which reveals a monotonic two-fold decrease in μ Hall on cooling from 190 to 30 K, demonstrating that μ Hall ( T ) is not yet phonon-limited. We, in fact, observe weak carrier freeze-out, an Arrhenius plot of p ( T ) yielding activation energies as low as 2.5 meV ( Supplementary Fig. S4 ). 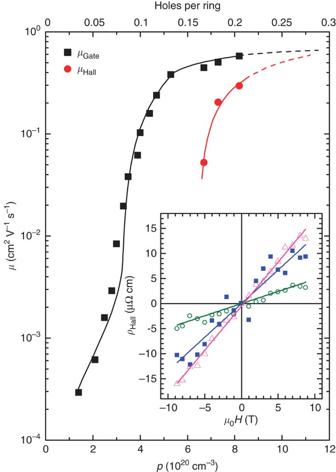Figure 5: Observation of the Hall effect. Hole density dependence of the 190 K mobility (μ) extracted from the integrated charge and measured via the Hall effect. Inset: Hall resistivity (ρHall) versusμ0Hfor three different gate voltages at 190 K; −1.00 V (red triangles), −0.95 V (blue squares) and −0.90 V (green circles). The zero field Hall resistivity has been subtracted from the data. The solid lines are linear fits. Figure 5: Observation of the Hall effect. Hole density dependence of the 190 K mobility ( μ ) extracted from the integrated charge and measured via the Hall effect. Inset: Hall resistivity ( ρ Hall ) versus μ 0 H for three different gate voltages at 190 K; −1.00 V (red triangles), −0.95 V (blue squares) and −0.90 V (green circles). The zero field Hall resistivity has been subtracted from the data. The solid lines are linear fits. Full size image We believe that the picture that emerges from this work is quite clear. At mobilities approaching 1 cm 2 V −1 s −1 conductive polymer thin film transistors can apparently be doped to the verge of the crossover from a strongly non-adiabatic VRH regime to an adiabatic, diffusive, band-like transport regime, where a Hall signal can be detected for the first time. This occurs despite the identification of a potential limitation of electrochemical doping, where doping-induced disorder limits carrier wavefunction delocalization. The results indicate that truly diffusive band-like transport is likely within reach in low-temperature solution-processed plastic transistors, an advance that would open up myriad opportunities in organic electronics. Device fabrication The raw materials consisted of (a) P3HT (Rieke Metals, measured M n of 23 kDa); (b) an ion gel ink composed of a mixture of 1.5 wt% poly(styrene- b -methylmethacrylate- b -styrene (PS-PMMA-PS) triblock copolymer ( M n =13–65–13 kDa, polydispersity 1.3), 8.5 wt% 1-ethyl-3-methylimidazolium bis(trifluoro-methylsulfonyl) imide ((EMIM)(TFSI)) ionic liquid (Merck), and 90 wt% ethyl acetate; and (c) PEDOT:PSS ink (PH 500, 1–1.4 wt% polymer in H 2 O, from H.C. Stark), diluted with 10 vol% ethylene glycol to enhance conductivity. To fabricate 4-probe 500 × 500 μm devices, Cr (2.5 nm)/Au (25 nm) bottom electrodes were first photolithographically patterned on Kapton substrates (Dupont) of thickness 50 μm. P3HT was then spin-coated from a chloroform solution (6 mg ml −1 ) to a thickness of 60 nm. The root-mean-square roughness of the bare Kapton substrates and the P3HT film were found to be ~1 nm over a 5 × 5-μm area by atomic force microscopy (see Supplementary Fig. S1 ). The P3HT layer was then manually patterned using a chloroform-soaked swab. The ion gel and gate electrodes (5 and 1 μm thick, respectively) were subsequently printed using a commercial aerosol-jet system (Optomec, Inc., see ref. 18 for details), and the device was baked in a N 2 -filled glove box for 3 h at 110 °C. Measurement details Electronic transport measurements were performed in He vapour in a commercial cryostat/superconducting magnet system wired with cryogenic sub-miniature coaxial cable. Isothermal transfer curves were measured DC, with a voltage sweep rate of 50 mV s −1 . Most of the temperature-dependent resistivity measurements were also performed DC, using a source/measure unit to source current, and a high-input-impedance, high-sensitivity multimeter to measure voltage. To improve signal-to-noise ratio in Hall and magnetoresistance measurements, a 13.7 Hz AC excitation was employed (using an AC resistance bridge), in the cases where the two-terminal resistance was ~10 kΩ or lower. In all cases, extensive checks were made for self-heating and Ohmic response, particularly at low temperatures. Additional information on the methods employed for the transport measurements and their analysis is provided in Supplementary Figs S2–S5 . How to cite this article: Wang, S. et al . Hopping transport and the Hall effect near the insulator–metal transition in electrochemically gated poly(3-hexylthiophene) transistors. Nat. Commun. 3:1210 doi: 10.1038/ncomms2213 (2012).